Increased CRF signalling in a ventral tegmental area-interpeduncular nucleus-medial habenula circuit induces anxiety during nicotine withdrawal Increased anxiety is a prominent withdrawal symptom in abstinent smokers, yet the neuroanatomical and molecular bases underlying it are unclear. Here we show that withdrawal-induced anxiety increases activity of neurons in the interpeduncular intermediate (IPI), a subregion of the interpeduncular nucleus (IPN). IPI activation during nicotine withdrawal was mediated by increased corticotropin releasing factor (CRF) receptor-1 expression and signalling, which modulated glutamatergic input from the medial habenula (MHb). Pharmacological blockade of IPN CRF1 receptors or optogenetic silencing of MHb input reduced IPI activation and alleviated withdrawal-induced anxiety; whereas IPN CRF infusion in mice increased anxiety. We identified a mesointerpeduncular circuit, consisting of ventral tegmental area (VTA) dopaminergic neurons projecting to the IPN, as a potential source of CRF. Knockdown of CRF synthesis in the VTA prevented IPI activation and anxiety during nicotine withdrawal. These data indicate that increased CRF receptor signalling within a VTA–IPN–MHb circuit triggers anxiety during nicotine withdrawal. Smoking is the primary cause of preventable mortality in the world [1] . Nicotine withdrawal symptoms are major factors that contribute to the low success rates of quit attempts [2] , [3] , [4] . In particular, increased anxiety during nicotine cessation is a prominent affective withdrawal symptom, yet little is known regarding the neuroanatomical bases of anxiety during nicotine withdrawal or the neuroadaptations induced by chronic nicotine that trigger the anxiogenic effects of nicotine withdrawal. While the vast majority of studies on nicotine dependence in animal models have focused on the traditional mesocorticolimbic ‘reward’ circuitry of the central nervous system (CNS) [5] , [6] , [7] , [8] , [9] , a much more understudied circuit that may be critical for nicotine dependence—the habenulo-interpeduncular pathway [10] , [11] , [12] —has recently gained attention. This circuit consists of the habenula (Hb), a small, epithalamic structure, that can be divided into medial (MHb) and lateral (LHb) sub-regions [13] . The LHb projects to the rostromedial tegmental nucleus that is involved in the modulation of dopamine (DA) release from the substantia nigra pars compacta and ventral tegmental area (VTA) [14] , [15] , [16] , [17] , [18] , [19] , while the MHb projects to the interpeduncular nucleus (IPN) which, in turn, prominently projects to the median and dorsal raphe nuclei, serotonergic-rich regions that modulate emotional states such as anxiety [20] . Recent data indicate that the Hb–IPN axis controls nicotine intake in rodents and plays a role in the acute aversive effects of high nicotine doses [10] , [21] . In addition, activation of GABAergic neurons within the IPN triggers somatic withdrawal symptoms in nicotine-dependent mice, suggesting that the IPN is a critical circuit for the expression of physical symptoms of nicotine withdrawal [22] . However, the role of the IPN in the affective symptoms of withdrawal, such as anxiety, remains to be elucidated. It has been hypothesized that withdrawal from chronic nicotine, as well as other drugs of abuse such as cocaine, may trigger overactivation of the stress circuitry in the CNS [23] , [24] . One of the predominant stress modulators in this circuitry is corticotropin releasing factor (CRF), a 41amino-acid neuropeptide that binds to and activates its cognate G-protein-coupled receptors, CRF type 1 (CRF1) and CRF type 2 (CRF2) [25] . The precise network and mechanistic basis for the CRF system in the anxiogenic effects of nicotine withdrawal is largely unknown. Here we show that CRF inputs from the VTA and glutamatergic inputs from the MHb converge onto a subset of IPN neurons to regulate anxiety during nicotine withdrawal via CRF1 receptor activation. To induce nicotine dependence, we passively exposed male C57BL/6J mice to nicotine by adding it to their drinking water. Drinking water was laced with 200 μg ml −1 nicotine tartrate, a dose used in previous studies to induce dependence, and sweetened with 0.3% saccharin to increase palatability [26] , [27] . Control mice were given drinking water containing an equal dose of tartrate and saccharin. After 4 weeks of exposure to nicotine through their drinking water, mice had an average blood serum concentration of 941.8±126.1 ng ml −1 cotinine (a biomarker of nicotine exposure, n =8); whereas control mice had a concentration of 1.54±0.1 ng ml −1 cotinine ( n =4). All nicotine-treated mice had at least 300 ng ml −1 serum cotinine, consistent with concentrations achieved by heavy smokers [28] . The IPN is a substrate of anxiety during nicotine withdrawal To test the hypothesis that the IPN is involved in the anxiogenic effects of nicotine withdrawal, we implanted cannulas targeting the IPN and infused mecamylamine (1 and 3 μg) into this area prior to measuring anxiety behaviours in mice that had received a 4- to 6-week exposure to control or nicotine solution ( Fig. 1 ). We evaluated anxiety-like behaviour via elevated plus maze (EPM) and the marble-burying test (MBT) [29] , [30] . In the MBT, two-way analysis of variance (ANOVA) indicated a significant main effect of drug infusion (F 2,70 =13.28, P <0.0001) and chronic treatment (F 1,70 =26.87, P <0.001), and a significant interaction (F 2,70 =9.40, P =0.0002). Mecamylamine infusion did not significantly affect marble burying in nicotine-naive mice compared with a saline infusion. However, post hoc analysis revealed that chronic nicotine-treated mice receiving a 1 or 3 μg mecamylamine infusion buried significantly more marbles compared with either chronic nicotine-treated mice receiving a saline IPN infusion ( Fig. 1a ) or nicotine-naive mice receiving mecamylamine infusions ( Fig. 1a ). In the EPM, two-way ANOVA revealed that there was a significant main effect of IPN infusion (F 2,59 =3.33, P =0.043) and chronic treatment (F 1,59 =7.76, P =0.007), and a significant interaction (F 2,59 =4.85, P =0.011). Mecamylamine infusion into the IPN of nicotine-naive mice did not affect time spent in the open arms compared with a saline infusion. In nicotine-dependent animals, IPN infusion of both mecamylamine doses significantly reduced time spent in the open arms of the EPM ( Fig. 1b ) compared with a saline infusion. Importantly, IPN infusion of saline or mecamylamine did not affect total arm entries in either group of animals, indicating results were not influenced by non-specific effects of infusion on locomotor activity ( Fig. 1c ). Cannula placements were verified in each mouse by analysing cresyl violet staining and also by infusing DiI into the brain before tissue harvesting ( Supplementary Fig. 1 ). To test the hypothesis that the effect of mecamylamine on anxiety in nicotine-dependent animals was specific to the IPN, we implanted cannulas targeting neighbouring brain regions lateral and caudal to the IPN, the VTA and median raphe (MnR), respectively. Infusion of mecamylamine in either the VTA or MnR had no significant effects on behaviour in nicotine-dependent mice in the MBT or EPM ( Supplementary Fig. 2a–c and Supplementary Fig. 3a–c ). As with IPN infusions, cannula placements for the VTA and MnR infusions were verified ( Supplementary Fig. 2d, e and Supplementary Fig. 3d, e , respectively). These data indicate that blockade of IPN nicotinic acetylcholine receptors (nAChRs) in nicotine-dependent, but not nicotine-naive, mice was sufficient to precipitate anxiety-like behaviour. 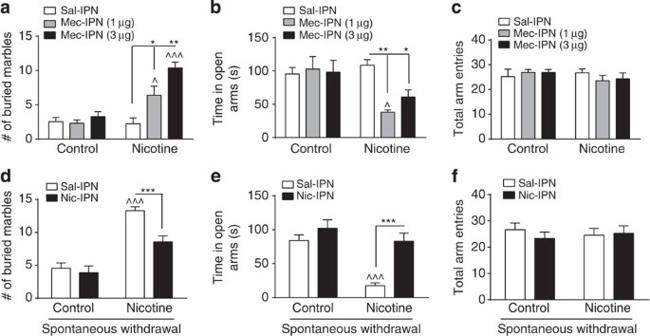Figure 1: The IPN is a neuroanatomical substrate of anxiety during nicotine withdrawal. (a) Average number of marbles buried in control and chronic nicotine-treated mice after saline (n=13 mice per group) or mecamylamine (1 μg,n=13 mice per group and 3 μg,n=12 and 13, respectively) infusion into the IPN. (b) Average time spent in the open arms of the EPM in control or chronic nicotine-treated mice after an IPN infusion of saline (n=10 mice per group) or mecamylamine (1 μg,n=10 and 8 mice, respectively, and 3 μg,n=10 mice per group). (c) Average total arm entries in control or chronic nicotine-treated animals after IPN infusion of saline or mecamylamine from mice inb. (d) Average number of marbles buried in control and chronic nicotine-treated mice after saline (n=11 and 10, respectively) or nicotine (100 ng,n=9 mice per group) infusion into the IPN. Behaviour was measured 24 h after control or nicotine solution was replaced with water. (e) Average time spent in the open arms of the EPM in control or chronic nicotine-treated mice during spontaneous withdrawal after an IPN infusion of saline (n=15 and 11, respectively) or nicotine (n=9 and 10, respectively). (f) Average total arm entries in withdrawn control or chronic nicotine-treated animals after IPN infusion of saline or nicotine from mice ine. Data are expressed as mean±s.e.m. Two-way ANOVA, Bonferronipost hoctest. *P<0.05, **P<0.01, ***P<0.001 for saline compared with drug infusion within groups. ^P<0.05, ^^^P<0.001 for drug infusion in nicotine-treated animals compared with infusions in control-treated animals. Figure 1: The IPN is a neuroanatomical substrate of anxiety during nicotine withdrawal. ( a ) Average number of marbles buried in control and chronic nicotine-treated mice after saline ( n =13 mice per group) or mecamylamine (1 μg, n =13 mice per group and 3 μg, n =12 and 13, respectively) infusion into the IPN. ( b ) Average time spent in the open arms of the EPM in control or chronic nicotine-treated mice after an IPN infusion of saline ( n =10 mice per group) or mecamylamine (1 μg, n =10 and 8 mice, respectively, and 3 μg, n =10 mice per group). ( c ) Average total arm entries in control or chronic nicotine-treated animals after IPN infusion of saline or mecamylamine from mice in b . ( d ) Average number of marbles buried in control and chronic nicotine-treated mice after saline ( n =11 and 10, respectively) or nicotine (100 ng, n =9 mice per group) infusion into the IPN. Behaviour was measured 24 h after control or nicotine solution was replaced with water. ( e ) Average time spent in the open arms of the EPM in control or chronic nicotine-treated mice during spontaneous withdrawal after an IPN infusion of saline ( n =15 and 11, respectively) or nicotine ( n =9 and 10, respectively). ( f ) Average total arm entries in withdrawn control or chronic nicotine-treated animals after IPN infusion of saline or nicotine from mice in e . Data are expressed as mean±s.e.m. Two-way ANOVA, Bonferroni post hoc test. * P <0.05, ** P <0.01, *** P <0.001 for saline compared with drug infusion within groups. ^ P <0.05, ^^^ P <0.001 for drug infusion in nicotine-treated animals compared with infusions in control-treated animals. Full size image Next, we implanted cannulas targeting the IPN in nicotine-treated mice and then replaced nicotine-drinking bottles with water bottles to induce spontaneous withdrawal. Anxiety-like behaviours were measured 24 h after nicotine bottle replacement. Before measuring anxiety behaviours during spontaneous withdrawal, we infused the IPN with either saline or 100 ng nicotine. In the MBT, two-way ANOVA indicated a significant main effect of drug infusion (F 1,35 =10.13, P =0.0031) and chronic treatment (F 1,35 =62.56, P <0.0001) and a significant interaction (F 1,35 =5.80, P =0.021). Post hoc analysis revealed that mice undergoing spontaneous nicotine withdrawal and infused with saline in the IPN before testing, buried significantly more marbles compared with control mice infused with saline ( Fig. 1d ), indicating increased anxiety-like behaviour during spontaneous nicotine withdrawal. In addition, nicotine infusion into the IPN of nicotine-dependent animals undergoing spontaneous withdrawal significantly reduced the number of marbles buried compared with withdrawn animals given a saline IPN infusion ( Fig. 1d ). Nicotine infusion into the IPN did not significantly affect the number of marbles buried in control mice compared with saline. In the EPM, two-way ANOVA revealed a significant main effect of drug infusion (F 1,41 =19.21, P <0.0001), chronic treatment (F 1,41 =20.3, P <0.0001) and a significant interaction (F 1,41 =6.21, P =0.0169). Nicotine infusion in the IPN had no effect on time spent in the open arms of the EPM in control mice. However, nicotine infused in the IPN significantly increased time spent in the open arms in chronic, nicotine-treated animals undergoing withdrawal compared with saline infusion ( Fig. 1e ). Neither saline nor nicotine infusion influenced the total number of EPM arm entries ( Fig. 1f ). These data indicate that nicotine infused into the IPN alleviated anxiety during nicotine withdrawal, further supporting a role for the IPN in nicotine withdrawal-induced anxiety. CRF1 receptor signalling in withdrawal-induced anxiety Does the IPN express CRF and its cognate receptors? To address this question, we analysed mRNA expression within the IPN. The IPN robustly expresses CRF1 receptor mRNA and, to a lesser extent, CRF2 receptor mRNA ( Table 1 ), consistent with previous reports [31] . In addition, expression of CRF mRNA itself was detected. To determine if CRF has a behavioural role within the IPN, we infused 50 ng CRF into the IPN of control and chronic nicotine-treated mice ( Fig. 2a–c ). In the MBT, two-way ANOVA revealed a significant main effect of drug infusion (F 1,46 =8.62, P =0.0052), chronic treatment (F 1,46 =11.02, P =0.0018) and a significant interaction (F 1,46 =4.79, P =0.034). In nicotine-naive mice, CRF failed to significantly modulate marble burying compared with a saline infusion ( Fig. 2a ). However, CRF infusion in nicotine-dependent mice significantly increased marble burying compared with saline- and CRF-infused nicotine-naive animals. In the EPM, two-way ANOVA indicated a significant main effect of drug infusion (F 1,58 =33.01, P <0.0001), chronic treatment (F 1,58 =5.45, P =0.023) and a significant interaction (F 1,58 =4.99, P =0.020). CRF infusion decreased open arm time in both control and nicotine-dependent animals compared with saline infusions with a larger decrease in nicotine-dependent mice ( Fig. 2b ). CRF infusion did not affect total arm entries of the EPM in control or nicotine-dependent mice. Table 1 Quantitative gene expression of CRF1, CRF2 and CRF in the IPN. 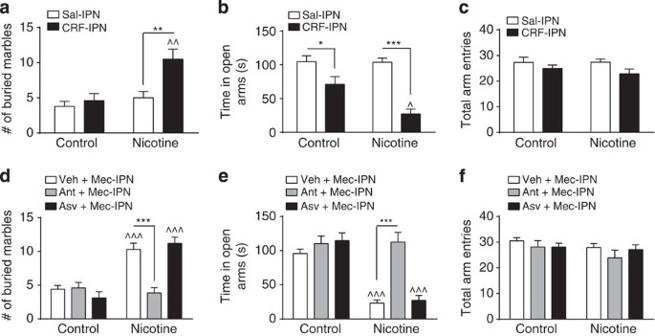Figure 2: CRF receptor signalling in the IPN mediates anxiety during nicotine withdrawal. (a) Average number of marbles buried in control and chronic nicotine-treated, non-withdrawn mice after infusion of saline (n=14 and 9, respectively) or 50 ng (n=17 and 10, respectively) CRF into the IPN. (b) Average time spent in the open arms of the EPM in control or chronic nicotine-treated, non-withdrawn mice after an IPN infusion of saline (n=20 and 15 mice, respectively) or 50 ng (n=17 and 10, respectively) CRF into the IPN. (c) Average total arm entries in control or chronic nicotine-treated, non-withdrawn animals after IPN infusion of saline or CRF fromb. (d) Average number of marbles buried in control and chronic nicotine-treated mice after preinfusion of Vehicle (Veh, 5% DMSO in saline,n=10 mice per group), the CRF1 receptor antagonist, antalarmin (1 μg,n=12 and 13, respectively), or the CRF2 receptor antagonist, antisauvagine 30 (2 μg,n=10 mice per group) before an infusion of mecamylamine (to precipitate withdrawal, 3 μg,) into the IPN. (e) Average time spent in the open arms of the EPM in control or chronic nicotine-treated mice after an IPN preinfusion of saline (n=10 mice per group), antalarmin (n=9 and 10) or antisauvagine 30 (n=10 mice per group) before an infusion of mecamylamine. (f) Average total arm entries in control or chronic nicotine-treated animals after IPN infusions as above. Data are expressed as mean±s.e.m. Two-way ANOVA, Bonferronipost hoctest. *P<0.05, **P<0.01, ***P<0.001 for saline compared with drug infusion within groups. ^P<0.05, ^^P<0.01, ^^^P<0.001 for drug infusion in nicotine-treated animals compared with infusions in control-treated animals. Full size table Figure 2: CRF receptor signalling in the IPN mediates anxiety during nicotine withdrawal. ( a ) Average number of marbles buried in control and chronic nicotine-treated, non-withdrawn mice after infusion of saline ( n =14 and 9, respectively) or 50 ng ( n =17 and 10, respectively) CRF into the IPN. ( b ) Average time spent in the open arms of the EPM in control or chronic nicotine-treated, non-withdrawn mice after an IPN infusion of saline ( n =20 and 15 mice, respectively) or 50 ng ( n =17 and 10, respectively) CRF into the IPN. ( c ) Average total arm entries in control or chronic nicotine-treated, non-withdrawn animals after IPN infusion of saline or CRF from b . ( d ) Average number of marbles buried in control and chronic nicotine-treated mice after preinfusion of Vehicle (Veh, 5% DMSO in saline, n =10 mice per group), the CRF1 receptor antagonist, antalarmin (1 μg, n =12 and 13, respectively), or the CRF2 receptor antagonist, antisauvagine 30 (2 μg, n =10 mice per group) before an infusion of mecamylamine (to precipitate withdrawal, 3 μg,) into the IPN. ( e ) Average time spent in the open arms of the EPM in control or chronic nicotine-treated mice after an IPN preinfusion of saline ( n =10 mice per group), antalarmin ( n =9 and 10) or antisauvagine 30 ( n =10 mice per group) before an infusion of mecamylamine. ( f ) Average total arm entries in control or chronic nicotine-treated animals after IPN infusions as above. Data are expressed as mean±s.e.m. Two-way ANOVA, Bonferroni post hoc test. * P <0.05, ** P <0.01, *** P <0.001 for saline compared with drug infusion within groups. ^ P <0.05, ^^ P <0.01, ^^^ P <0.001 for drug infusion in nicotine-treated animals compared with infusions in control-treated animals. Full size image To test the hypothesis that chronic nicotine regulates expression of the CRF-CRF receptor pathway in the IPN, we quantified gene expression of CRF, CRF1 and CRF2 receptors in the IPN of control mice and mice that received chronic nicotine. When compared with nicotine-naive mice, chronic nicotine-treated animals displayed a significant, upregulation of CRF1, but not CRF2 receptor mRNA within the IPN ( Table 1 ). To test the hypothesis that signalling specifically through CRF1 receptors is involved in the anxiogenic effects of nicotine withdrawal, we preinfused CRF1 or CRF2 receptor antagonists into the IPN before mecamylamine infusion. In one group of mice, we preinfused the CRF1 receptor-selective antagonist, antalarmin [32] , while another group received the CRF2 receptor antagonist, antisauvagine-30 (ref. 33 ). Control mice received vehicle before mecamylamine alone. In the MBT, two-way ANOVA indicated a significant main effect of drug infusion (F 2,59 =9.49, P =0.0003) and chronic treatment (F 1,59 =41.95, P <0.0001) and a significant interaction (F 2,59 =16.17, P <0.0001). An IPN infusion of mecamylamine increased the number of marbles buried in chronic nicotine-treated animals and this effect was significantly reduced by a preinfusion of antalarmin ( Fig. 2d ) but not antisauvagine-30. Similarly, with respect to open arm time in the EPM, two-way ANOVA revealed significant main effect of chronic treatment (F 1,53 =45.22, P <0.0001), infusion (F 2,53 =15.91, P <0.0001) and a significant interaction (F 2,53 =12.33, P <0.0001). Mecamylamine infusion reduced time spent in the open arms in nicotine-treated mice and this was significantly increased by an IPN preinfusion of antalarmin ( Fig. 2e ), but not antisauvagine-30. Drug infusion had no effect on the number of total arm entries in any group ( Fig. 2f ). These data implicate a role for CRF1 but not CRF2 receptor signalling in nicotine withdrawal-induced anxiety. Nicotine withdrawal activates IPI neurons via CRF1 receptors The IPN is divided into distinct sub-regions including rostral, intermediate, lateral and central (IPR, IPI, IPL and IPC, respectively) [20] . We challenged nicotine-dependent and nicotine-naive mice with mecamylamine (3 mg kg −1 , intraperitoneal (i.p.)). Brains were collected 90 min post-injection, sliced and immunolabeled with c-Fos [34] , a marker of neuronal activation ( Fig. 3a ). Previously we demonstrated that activation of GABAergic neurons within the IPR triggers somatic but not affective symptoms [22] . Thus, we focused analysis on the ventral portion of the IPN containing the IPI, IPL and IPC. In chronic, nicotine-treated mice, mecamylamine activated a discrete population of neurons located within the IPI ( Fig. 3a ). To test the hypothesis that activation was mediated by CRF1 receptors, we preinjected control and nicotine-treated mice with antalarmin (10 mg kg −1 , i.p.) [35] and counted the number of c-Fos-immunopositive neurons within the IPI. Two-way ANOVA revealed a significant main effect of chronic treatment (F 1,12 =27.25, P =0.0002), preinjection (F 1,12 =16.25, P =0.0017) and a significant interaction (F 1,12 =5.783, P =0.0332). Mecamylamine significantly increased the number of c-Fos immunopositive neurons within the IPI of chronic nicotine-treated animals compared with control animals ( Fig. 3b ). In addition, antalarmin preinjection significantly reduced the number of c-Fos immunopositive neurons in the IPI during mecamylamine-precipitated nicotine withdrawal ( Fig. 3b ). As with IPN infusion of antalarmin, systemic delivery of antalarmin reduced anxiety-like behaviour in mice undergoing mecamylamine-precipitated nicotine withdrawal ( Supplementary Fig. 4 ). We next tested whether neurons within the IPI express the CRF1 receptor. We performed fluorescent in situ hybridization (FISH) to detect CRF1 receptor mRNA in the IPN. Interestingly, CRF1 receptor mRNA is primarily localized to the IPI of the ventral IPN ( Fig. 3c ). To determine if CRF activates these neurons, we infused CRF into the IPN and combined FISH for visualization of CRF1 receptor mRNA expression with immunohistochemistry to detect c-Fos induction in the IPI. CRF infusion induced c-Fos expression specifically in the IPI. CRF1 receptor mRNA was also detected in the majority of c-Fos immunopositive neurons of the IPI ( Fig. 3d ). Finally, we confirmed that CRF1 receptor gene expression was upregulated in nicotine-dependent, compared to nicotine-naive, mice, specifically in laser-dissected ventral IPN ( Table 1 ). Together, these data indicate that CRF activates IPI neurons through CRF1 receptor signalling and this signalling is upregulated with chronic nicotine exposure. 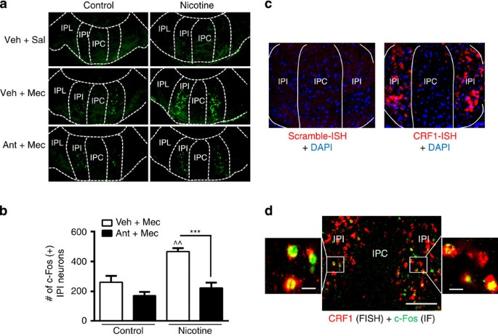Figure 3: Mecamylamine-precipitated withdrawal activates neurons within the IPI of the IPN through a CRF1 receptor-dependent mechanism. (a) Photomicrographs from coronal sections immunolabeled for c-Fos (green). Sections are taken from control or chronic nicotine-treated mice given i.p. injections of saline, mecamylamine (Mec, 3 mg kg−1) or antalarmin (Ant, 10 mg kg−1) before mecamylamine as indicated in the left-hand column. IPN sub-regions are indicated by dotted lines. (b) Each bar graph represents the average total number of c-Fos(+) IPI neurons after a mecamylamine i.p. injection or an injection of antalarmin 15 min before mecamylamine in control-treated (n=4 mice per treatment, 16 slices per mouse) or chronic nicotine-treated mice (n=3 and 5 mice per treatment, 16 slices per mouse). (c) Photomicrograph from representative coronal sections after FISH with a control (left) or CRF1 receptor probe. Note a robust CRF1 receptor signal is predominantly localized to the IPI sub-region of the IPN. (d) Photomicrograph of coronal sections from chronic nicotine-treated mice given a CRF infusion (300 ng) into the IPN. Sections are double-labelled for CRF1 receptor mRNA (using FISH, red) and c-Fos protein (using immunohistochemistry, green). Merged sections imaged at 10 × magnification are shown (middle). Scale bar: 200 μm. Outside sections shown at 63 × magnification illustrate localization of c-Fos in CRF1 receptor-expressing IPI neurons. Scale bar: 20 μm. Data are expressed as mean±s.e.m. Two-way ANOVA, Bonferronipost hoctest. ***P<0.001 compared with saline preinjection within groups. ^^P<0.01 chronic nicotine-treated compared with control-treated mice. Figure 3: Mecamylamine-precipitated withdrawal activates neurons within the IPI of the IPN through a CRF1 receptor-dependent mechanism. ( a ) Photomicrographs from coronal sections immunolabeled for c-Fos (green). Sections are taken from control or chronic nicotine-treated mice given i.p. injections of saline, mecamylamine (Mec, 3 mg kg −1 ) or antalarmin (Ant, 10 mg kg −1 ) before mecamylamine as indicated in the left-hand column. IPN sub-regions are indicated by dotted lines. ( b ) Each bar graph represents the average total number of c-Fos(+) IPI neurons after a mecamylamine i.p. injection or an injection of antalarmin 15 min before mecamylamine in control-treated ( n =4 mice per treatment, 16 slices per mouse) or chronic nicotine-treated mice ( n =3 and 5 mice per treatment, 16 slices per mouse). ( c ) Photomicrograph from representative coronal sections after FISH with a control (left) or CRF1 receptor probe. Note a robust CRF1 receptor signal is predominantly localized to the IPI sub-region of the IPN. ( d ) Photomicrograph of coronal sections from chronic nicotine-treated mice given a CRF infusion (300 ng) into the IPN. Sections are double-labelled for CRF1 receptor mRNA (using FISH, red) and c-Fos protein (using immunohistochemistry, green). Merged sections imaged at 10 × magnification are shown (middle). Scale bar: 200 μm. Outside sections shown at 63 × magnification illustrate localization of c-Fos in CRF1 receptor-expressing IPI neurons. Scale bar: 20 μm. Data are expressed as mean±s.e.m. Two-way ANOVA, Bonferroni post hoc test. *** P <0.001 compared with saline preinjection within groups. ^^ P <0.01 chronic nicotine-treated compared with control-treated mice. Full size image CRF1 receptor activation modulates glutamatergic signalling We next measured frequencies and amplitudes of sEPSCs from IPI neurons of mouse IPN slices. We identified at least two distinct neuronal populations within the IPI, which we denote Type 1 and Type 2 ( Supplementary Fig. 5 ). Type 1 and Type 2 neurons were discernable based on biophysical parameters including resting membrane potential (−62.5±0.59 mV, n =68 and −76.1±0.97 mV, n =22, respectively; t 88 =11.44, P <0.0001, two-tailed t -test), membrane capacitance (29.9±1.6 pF, n =64 and 14.8±1.4 pF, n =21, respectively; t 83 =5.17, P <0.0001, two-tailed t -test), voltage-sag on hyperpolarization and hyperpolarization-activated currents ( Supplementary Fig. 5a–c ). To determine if Type 1 and/or 2 IPI neurons functionally express the CRF1 receptor, we measured sEPSCs in response to CRF. Bath application of CRF did not significantly modulate sEPSC frequency or amplitude in Type 1 neurons ( Fig. 4a–c , Supplementary Table 1 ); whereas CRF significantly and reversibly increased both sEPSC frequency and amplitude in Type 2 neurons ( Fig. 4d–f , Supplementary Table 1 ). Single-neuron RT–PCR detected CRF1 receptor transcripts in 100% of Type 2 neurons and ∼ 30% of Type 1 neurons ( Supplementary Fig. 5e, f ). To determine if the increased sEPSC amplitudes in Type 2 neurons could be caused by increased activation of CRF1 receptors, which are known to modulate glutamate-mediated NMDA receptor current amplitudes and glutamate release [36] , [37] , [38] , we measured the effect of antalarmin on sEPSC frequency and amplitude in IPI neurons from nicotine-withdrawn animals. In Type 1 neurons from withdrawn animals, antalarmin did not significantly modulate sEPSC frequency or amplitude ( Fig. 4g–i , Supplementary Table 1 ). In contrast, antalarmin significantly and reversibly reduced both sEPSC frequency and amplitude in Type 2 neurons in nicotine-withdrawn animals ( Fig. 4j–l , Supplementary Table 1 ). In Type 2 neurons from withdrawn slices, CRF was able to modestly increase sEPSC frequency and amplitude suggesting that antalarmin was blocking activation of CRF1 receptors by CRF release ( Supplementary Fig. 6a–c ). To determine if CRF in Type 2 neurons directly modulates NMDA receptors, we measured electrically evoked NMDA currents in the absence or presence of CRF in slices from both nicotine-naive and nicotine-dependent mice. In control slices, CRF increased the amplitude of evoked NMDA currents. Potentiation was significantly greater in slices from nicotine-dependent mice and reduced in the presence of antalarmin ( Supplementary Fig. 6d,e ). 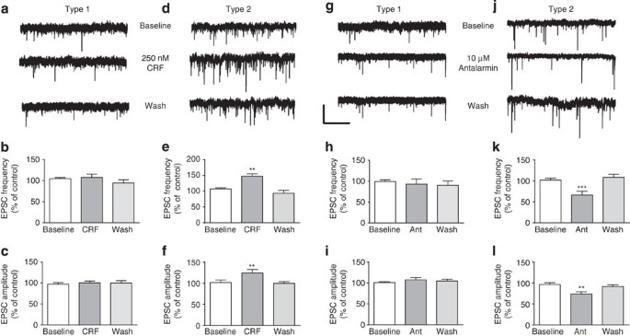Figure 4: CRF modulates glutamatergic activity in a subset of IPI neurons. Representative whole-cell voltage clamp recordings from Type 1 (a) and Type 2 (d) neurons within the IPI in response to CRF. Average sEPSC frequency and amplitude at baseline, after a 5-min application of CRF, and after washout from Type 1 (b,c, respectively,n=8 neurons) and Type 2 (e,f, respectively: one-way ANOVAs with repeated measures: Frequency, F2, 12=19.2,P=0.0002; Amplitude, F2, 12=10.49,P=0.0023,n=7) IPI neurons. Representative whole-cell voltage clamp recordings from Type 1 (g) and Type 2 (j) nicotine-withdrawn IPI neurons in response to antalarmin. Average sEPSC frequency and amplitude at baseline, after a 5-min application of antalarmin, and after washout from Type 1 (h,i, respectively,n=8) and Type 2 (k,l, respectively: Frequency, F2, 14=17.22,P=0.0002; Amplitude, F2, 14=13.66,P=0.0005,n=8) IPI neurons. Neurons were recorded in slices from nicotine-dependent mice. Scale bar:y=20 pA,x=5 s. Data are expressed as mean±s.e.m. **P<0.01 and ***P<0.0001. Figure 4: CRF modulates glutamatergic activity in a subset of IPI neurons. Representative whole-cell voltage clamp recordings from Type 1 ( a ) and Type 2 ( d ) neurons within the IPI in response to CRF. Average sEPSC frequency and amplitude at baseline, after a 5-min application of CRF, and after washout from Type 1 ( b , c , respectively, n =8 neurons) and Type 2 ( e , f , respectively: one-way ANOVAs with repeated measures: Frequency, F 2, 12 =19.2, P =0.0002; Amplitude, F 2, 12 =10.49, P =0.0023, n =7) IPI neurons. Representative whole-cell voltage clamp recordings from Type 1 ( g ) and Type 2 ( j ) nicotine-withdrawn IPI neurons in response to antalarmin. Average sEPSC frequency and amplitude at baseline, after a 5-min application of antalarmin, and after washout from Type 1 ( h , i , respectively, n =8) and Type 2 ( k , l , respectively: Frequency, F 2, 14 =17.22, P =0.0002; Amplitude, F 2, 14 =13.66, P =0.0005, n =8) IPI neurons. Neurons were recorded in slices from nicotine-dependent mice. Scale bar: y =20 pA, x =5 s. Data are expressed as mean±s.e.m. ** P <0.01 and *** P <0.0001. Full size image To test the hypothesis that increased anxiety during nicotine withdrawal is indeed mediated by glutamatergic signalling in the IPN and activation of IPI neurons, we infused the NMDA receptor antagonist, AP5, or vehicle into the IPN before mecamylamine infusion in nicotine-dependent and nicotine-naive animals and measured anxiety-like behaviour and c-Fos expression ( Fig. 5 ). In the MBT, two-way ANOVA revealed a significant effect of chronic treatment (F 1,49 =11.46, P =0.0014), infusion (F 2,49 =5.21, P =0.0089) and a significant interaction (F 2,49 =7.15, P =0.0019). Saline, mecamylamine or preinfusion of either AP5 or vehicle did not significantly affect any measure of anxiety-like behaviour in nicotine-naive mice ( Fig. 5a ). However, in nicotine-dependent animals, an IPN infusion of mecamylamine increased the number of marbles buried compared with saline infusion ( Fig. 5a ). Preinfusion of AP5 significantly reduced this number. In the EPM, two-way ANOVA indicated a significant effect of chronic treatment (F 1,39 =4.62, P =0.038), infusion (F 1,39 =10.28, P =0.0027) and a significant interaction (F 1,39 =4.12, P =0.0491). In nicotine-dependent mice, mecamylamine decreased time spent in the open arms of the EPM compared with nicotine-naive animals, an effect reversed by preinfusion of AP5 but not saline ( Fig. 5b ). Drug infusions did not affect total arm entries in the EPM ( Fig. 5c ). Analysing neuronal activation ( Fig. 5d,e ), two-way ANOVA revealed a significant effect of chronic treatment (F 1,10 =30.31, P <0.0003), preinfusion (F 1,10 =48.00, P =0.0001), and an interaction (F 1,10 =18.09, P <0.01). Infusion of mecamylamine significantly increased the number of c-Fos immunopositive neurons in the IPI of nicotine-dependent animals compared to nicotine-naive mice. This increase was significantly reduced by a preinfusion of AP5 but not saline. 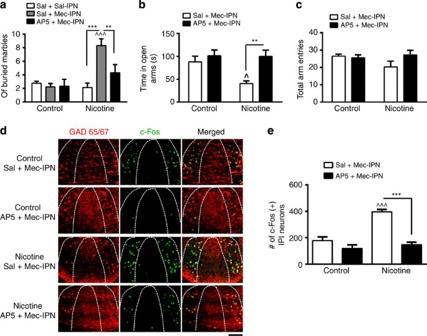Figure 5: Glutamatergic signalling in the IPN is critical for expression of anxiety-like behaviour during nicotine withdrawal. (a) Average number of marbles buried in control and chronic nicotine-treated mice after infusion of saline prior to saline (n=8 mice/group), saline prior to mecamylamine (3 μg,n=10 mice/group), or AP5 (0.3 μg) prior to mecamylamine (n=9 and 10, respectively) into the IPN. (b) Average time spent in the open arms of the EPM in control or chronic nicotine-treated mice after infusion of saline (n=12 mice/group) or AP5 (n=9 and 10, respectively) prior to mecamylamine into the IPN. (c) Average total arm entries in control or chronic nicotine-treated animals after infusion of saline or AP5 prior to mecamylamine from mice in panelb. (d) Representative IPI sections from control or chronic nicotine-treated mice after IPN infusion of Sal+Mec, or AP5+Mec. Sections were immunolabeled for GAD2/1 (red, left panels) and c-Fos (green, middle panels). Right panels depict merged signals. Scale bar: 100 μm. (e) Averaged total number of c-Fos immunopositive IPI neurons for each condition in paneld(control mice,n=3 mice/treatment, 16 slices/mouse; chronic nicotine-treated mice,n=4 mice/treatment, 16 slices/mouse). Data are expressed as mean±s.e.m. Two-way ANOVA, Bonferronipost hoctest. **P<0.01, ***P<0.001. ^P<0.05, ^^^P<0.001 for drug infusion in nicotine-treated animals compared to infusions in control-treated animals. Figure 5: Glutamatergic signalling in the IPN is critical for expression of anxiety-like behaviour during nicotine withdrawal. ( a ) Average number of marbles buried in control and chronic nicotine-treated mice after infusion of saline prior to saline ( n =8 mice/group), saline prior to mecamylamine (3 μg, n =10 mice/group), or AP5 (0.3 μg) prior to mecamylamine ( n =9 and 10, respectively) into the IPN. ( b ) Average time spent in the open arms of the EPM in control or chronic nicotine-treated mice after infusion of saline ( n =12 mice/group) or AP5 ( n =9 and 10, respectively) prior to mecamylamine into the IPN. ( c ) Average total arm entries in control or chronic nicotine-treated animals after infusion of saline or AP5 prior to mecamylamine from mice in panel b . ( d ) Representative IPI sections from control or chronic nicotine-treated mice after IPN infusion of Sal+Mec, or AP5+Mec. Sections were immunolabeled for GAD2/1 (red, left panels) and c-Fos (green, middle panels). Right panels depict merged signals. Scale bar: 100 μm. ( e ) Averaged total number of c-Fos immunopositive IPI neurons for each condition in panel d (control mice, n =3 mice/treatment, 16 slices/mouse; chronic nicotine-treated mice, n =4 mice/treatment, 16 slices/mouse). Data are expressed as mean±s.e.m. Two-way ANOVA, Bonferroni post hoc test. ** P <0.01, *** P <0.001. ^ P <0.05, ^^^ P <0.001 for drug infusion in nicotine-treated animals compared to infusions in control-treated animals. Full size image Silencing MHb–IPN inputs reduces anxiety during withdrawal To test the hypothesis that glutamatergic input from the MHb plays a role in IPI activation and anxiety during nicotine withdrawal, we selectively expressed halorhodopsin in MHb cholinergic/glutamatergic neurons to silence neurotransmission in mice undergoing nicotine withdrawal ( Fig. 6 ). Halorhodopsin (version 3.0) with an eYFP tag (eNpHR-eYFP) was expressed in the MHb of ChAT-cre mice using AAV2-mediated gene delivery of a plasmid containing eNpHR-eYFP in a double-floxed inverted open-reading frame ( Supplementary Fig. 7a ) [39] . Four weeks post-infection, robust eYFP signal was observed in ChAT-expressing neurons and terminals innervating the IPN, indicating proper localization to cholinergic MHb neurons ( Fig. 6a ). Light stimulation of voltage-clamped eNpHR-eYFP-positive neurons in MHb slices from eNpHR-eYFP-infected ChAT-cre mice elicited outward currents at a holding potential of −70 mV under voltage clamp and hyperpolarization under current clamp, markedly silencing action potential firing ( Supplementary Fig. 7b ), confirming that eNpHR-eYFP was expressed and functional in MHb cholinergic neurons. 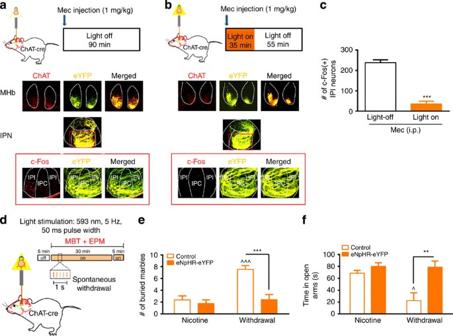Figure 6: IPN neurotransmission from the MHb is necessary for anxiety during nicotine withdrawal and activation of IPI neurons. In vivohalorhodopsin stimulation paradigm for analysis of the effect of MHb input on activation of IPI neurons during mecamylamine-precipitated nicotine withdrawal for light non-stimulated (a) and light-stimulated (b) mice expressing eNpHR-eYFP. Middle, photomicrographs from representative MHb and IPN coronal sections from each group illustrating eNpHR-eYFP expression (yellow). Bottom, representative coronal sections immunostained for c-Fos (left panel, red) and imaged for detection of eYFP (middle panel, yellow). Merged signals are depicted in the right-hand panel. (c) Average number of c-Fos immunopositive IPI neurons after mecamylamine-precipitated nicotine withdrawal in light non-stimulated (Light-off, 16 slices/mouse,n=4) and light-stimulated (Light on, 16 slices/mouse,n=5) mice expressing eNpHR-eYFP. ***P<0.001, two-tailed student’st-test. (d)In vivohalorhodopsin stimulation paradigm for analysis of the effect of MHb input on MBT and EPM assays during spontaneous nicotine withdrawal. (e) Number of marbles buried in nicotine-dependent, non-withdrawn (Nicotine) or nicotine-dependent, spontaneous withdrawn ChAT-cre mice (Withdrawal) expressing either control virus (Control,n=9) or halorhodopsin (eNpHR-eYFP,n=9 and 12, respectively). Behaviours in all groups were done during light stimulation. (e) Time spent on the open arms of the EPM in nicotine-dependent, non-withdrawn (Nicotine) or nicotine-dependent, spontaneous withdrawn ChAT-cre mice (Withdrawal) expressing either control virus (Control,n=8) or halorhodopsin (eNpHR-eYFP,n=9 and 12, respectively). Behaviours in all groups were done during light stimulation. (f) Total arm entries in the EPM for each group. Data are expressed as mean±s.e.m. Two-way ANOVA, Bonferronipost hoctest. **P<0.01, ***P<0.001 compared within groups. ^P<0.05, ^^^P<0.001 withdrawn, control virus-expressing mice compared to non-withdrawn control virus-expressing mice. Figure 6: IPN neurotransmission from the MHb is necessary for anxiety during nicotine withdrawal and activation of IPI neurons. In vivo halorhodopsin stimulation paradigm for analysis of the effect of MHb input on activation of IPI neurons during mecamylamine-precipitated nicotine withdrawal for light non-stimulated ( a ) and light-stimulated ( b ) mice expressing eNpHR-eYFP. Middle, photomicrographs from representative MHb and IPN coronal sections from each group illustrating eNpHR-eYFP expression (yellow). Bottom, representative coronal sections immunostained for c-Fos (left panel, red) and imaged for detection of eYFP (middle panel, yellow). Merged signals are depicted in the right-hand panel. ( c ) Average number of c-Fos immunopositive IPI neurons after mecamylamine-precipitated nicotine withdrawal in light non-stimulated (Light-off, 16 slices/mouse, n =4) and light-stimulated (Light on, 16 slices/mouse, n =5) mice expressing eNpHR-eYFP. *** P <0.001, two-tailed student’s t -test. ( d ) In vivo halorhodopsin stimulation paradigm for analysis of the effect of MHb input on MBT and EPM assays during spontaneous nicotine withdrawal. ( e ) Number of marbles buried in nicotine-dependent, non-withdrawn (Nicotine) or nicotine-dependent, spontaneous withdrawn ChAT-cre mice (Withdrawal) expressing either control virus (Control, n =9) or halorhodopsin (eNpHR-eYFP, n =9 and 12, respectively). Behaviours in all groups were done during light stimulation. ( e ) Time spent on the open arms of the EPM in nicotine-dependent, non-withdrawn (Nicotine) or nicotine-dependent, spontaneous withdrawn ChAT-cre mice (Withdrawal) expressing either control virus (Control, n =8) or halorhodopsin (eNpHR-eYFP, n =9 and 12, respectively). Behaviours in all groups were done during light stimulation. ( f ) Total arm entries in the EPM for each group. Data are expressed as mean±s.e.m. Two-way ANOVA, Bonferroni post hoc test. ** P <0.01, *** P <0.001 compared within groups. ^ P <0.05, ^^^ P <0.001 withdrawn, control virus-expressing mice compared to non-withdrawn control virus-expressing mice. Full size image To test the hypothesis that cholinergic/glutamatergic MHb inputs to the IPN were necessary for activation of the IPI during nicotine withdrawal, optic cannulas were implanted targeting the MHb terminal inputs to the IPN in chronic nicotine-treated AAV2 eNpHR-eYFP-infected ChAT-cre mice. IPI activation was induced by mecamylamine injection. Yellow light was delivered at 5 Hz with a 50 ms pulse width immediately post-injection for 30 min; whereas control animals had optic cannula implants but no light was delivered ( Fig. 6a, b ). Analysis of c-Fos expression in the IPI of each group revealed that silencing MHb inputs to the IPN significantly reduced IPI neuronal activation during mecamylamine-precipitated withdrawal compared to control ( t 7 =10.24, P <0.001, two-tailed t -test, Fig. 6c ). To test the hypothesis that silencing cholinergic/glutamatergic MHb–IPN inputs was sufficient to alleviate nicotine withdrawal-induced anxiety, ChAT-cre mice were infected with AAV2 eNpHR-eYFP or control virus (AAV2-ZsGreen) and optic cannulas were implanted targeting the MHb terminal inputs to the IPN in chronic nicotine-treated ChAT-cre mice ( Fig. 6d ). Before withdrawal, during chronic nicotine treatment, eNpHR-eYFP and control-virus mice were tested in the MBT and EPM assays. Baseline anxiety between groups was not significantly different in either MBT or EPM assays ( Supplementary Fig. 7c–e ). Mice were spontaneously withdrawn from nicotine and anxiety behaviours were measured 24 h after nicotine cessation. The effect of light stimulation during spontaneous withdrawal was measured in control and eNpHR-eYFP-infected animals. In addition, the effect of light stimulation on anxiety behaviour in nicotine-dependent, non-withdrawn mice was also measured. In the MBT, two-way ANOVA indicated a significant effect of withdrawal state (F 1,33 =13.38, P =0.0008), virus (F 1,33 =13.29, P =0.0009), and an interaction (F 1,33 =8.29, P =0.007) during light stimulation ( Fig. 6e ). Interestingly, nicotine-dependent, non-withdrawn mice expressing eNpHR-eYFP buried marbles similar to control-virus expressing mice; whereas nicotine-dependent mice undergoing withdrawal and expressing the control virus buried significantly more marbles compared with nicotine-dependent, non-withdrawn mice. The number of marbles buried was significantly reduced in nicotine-withdrawn mice expressing eNpHR-eYFP. Similarly, in the EPM assay, two-way ANOVA revealed a significant effect of withdrawal state (F 1,33 =12.05, P =0.0015), virus (F 1,33 =5.90, P =0.021) and an interaction (F 1,33 =5.26, P =0.028) during light stimulation ( Fig. 6f ). Time spent in the open arms of the EPM did not significantly differ in eNpHR-eYFP-expressing nicotine-dependent, non-withdrawn mice compared with control. However, time spent in the open arms of the EPM was significantly increased in eNpHR-eYFP mice undergoing nicotine withdrawal compared with control-virus expressing mice undergoing nicotine withdrawal ( Fig. 6f ). Total arm entries did not differ between groups ( Supplementary Fig. 7f ). To determine if rebound excitation between light pulses influenced anxiety-like behaviour during nicotine withdrawal, we selectively expressed channelrhodopsin with an eYFP tag (ChR2-eYFP) in MHb of ChAT-cre mice using AAV2-mediated gene delivery of a plasmid containing ChR2-eYFP in a double-floxed inverted open-reading frame [40] . Stimulation of MHb–IPN terminals in either nicotine-treated or withdrawn ChAT-cre mice did not reduce anxiety-like behaviour ( Supplementary Fig. 8 ). Together, these data indicate that input originating from the MHb is necessary for activation of the IPI and the anxiogenic effects of nicotine withdrawal. Meso-IPN circuit CRF regulates anxiety during withdrawal Recently, Grieder et al . [41] identified a population of VTA DAergic neurons that synthesize CRF, which may release in the IPN during nicotine withdrawal. Thus, we tested the hypothesis that CRF input into the IPI originates from the VTA. We selectively expressed ChR2-eYFP in the VTA of TH-cre mice ( Supplementary Fig. 9a ) as an anterograde label [42] . Four weeks post-infection, significant eYFP signal was observed in VTA neurons and light pulses in DAergic neurons elicited robust inward currents under voltage-clamp confirming proper localization ( Supplementary Fig. 9a ). Interestingly, eYFP signal was also detected in the ventral IPN including IPL, IPI and IPC sub-regions, but not in the IPR, revealing a mesointerpeduncular circuit ( Supplementary Fig. 9b ). To test the hypothesis that VTA CRF is critical for activation of IPI neurons during nicotine withdrawal and anxiety, we knocked down CRF expression in the VTA of C57Bl/6J mice using AAV2 delivery of the shRNAs used in Grieder et al . [41] . Knockdown of CRF in the VTA of shRNA-expressing mice resulted in a robust decrease in CRF gene expression ( ∼ 90%) compared with expression in control, scrambled shRNA (ctrlRNA)-expressing mice ( Fig. 7a , t 10 =11.1, P <0.0001, two-tailed t -test). VTA tyrosine hydroxlase expression did not significantly differ between control and shRNA-expressing mice ( Fig. 7a ). Infected animals were treated with chronic nicotine, challenged with mecamylamine to precipitate withdrawal and analysed for activation of IPI neurons ( Fig. 7b ). Two-way ANOVA indicated a significant effect of shRNA (F 1,9 =18.80, P <0.0019) and chronic treatment (F 1,9 =14.28, P <0.0044) on neuronal activation in the IPI. Post hoc analysis indicated that mecamylamine increased the number of c-Fos immunopositive neurons in nicotine-dependent mice compared with nicotine-naive animals expressing ctrlRNA ( Fig. 7b ). In contrast, IPI neuronal activation during withdrawal was significantly reduced in mice infected with CRF shRNA in the VTA compared with control-infected animals, suggesting CRF synthesized in the VTA is critical for IPI activation during withdrawal. As our data indicate that the CRF1 receptor is predominantly expressed in the IPI, whereas the IPR is also activated during withdrawal but is critical for somatic, not affective symptoms, we analysed activation of the IPR in shRNA-infected animals. While knockdown of CRF in the VTA significantly reduced activation of IPI neurons during withdrawal, activation of IPR neurons was unaffected ( Fig. 7c , significant effect of withdrawal state, F 1,8 =37.38, P =0.0003, but not shRNA). 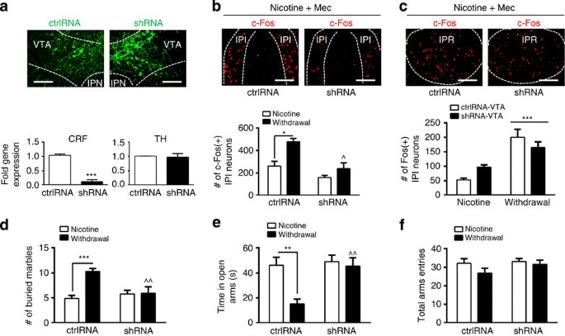Figure 7: Knockdown of CRF synthesis in the VTA reduces activity of IPI neurons and anxiety during nicotine withdrawal. (a) Representative photomicrographs from coronal sections containing the VTA (top). C57Bl/6J mouse brains were infected with control shRNA (ctrlRNA, left columns) or CRF shRNA (right columns) and were analysed for viral infection (green). Bottom, qRT-PCR comparing CRF (left) or TH (right) gene expression in ctrlRNA- and shRNA-infected VTA (n=6 mice/group). Gene expression was normalized to GAPDH. ***P<0.001, two-tailed student’st-test. (b) Top, photomicrographs depicting the IPI c-Fos pattern (green) induced by mecamylamine-precipitated withdrawal in chronic nicotine-treated mice expressing ctrlRNA (left) or CRF shRNA (right) in the VTA. Bottom, quantitative analysis of the number of IPI c-Fos immunopositive neurons during chronic nicotine before withdrawal and after mecamylamine-precipitated nicotine withdrawal from mice infected with ctrlRNA (n=3 and 4 mice/group, 14 slices/mouse) or CRF shRNAs (n=3 mice/group, 14 slices/mouse). (c) Top, photomicrographs depicting the IPR c-Fos pattern (green) induced by mecamylamine-precipitated withdrawal in chronic nicotine-treated mice expressing ctrlRNA (left) or CRF shRNA (right) in the VTA. Bottom, quantitative analysis of the number of IPR c-Fos immunopositive neurons during chronic nicotine before withdrawal and after mecamylamine-precipitated nicotine withdrawal from mice infected with ctrlRNA (n=3 and 4 mice/group) or CRF shRNAs (n=3). (d) Number of marbles buried in mice expressing ctrlRNA or CRF shRNA in the VTA during chronic nicotine exposure prior to withdrawal (n=15 and 18, respectively) and during spontaneous nicotine withdrawal (n=11 mice/group). (e) Time spent on the open arms of the EPM for mice expressing ctrlRNA or CRF shRNA in the VTA during chronic nicotine exposure prior to withdrawal (n=15 and 20, respectively) and during spontaneous nicotine withdrawal (n=11 mice/group). (f) Total arm entries in the EPM for each group in panele. Data are expressed as mean±s.e.m. Scale Bar: 100 μm. Two-way ANOVA, Bonferronipost hoctest. **P<0.01, **P<0.001. ^P<0.05, ^^P<0.01 for between group comparisons. Figure 7: Knockdown of CRF synthesis in the VTA reduces activity of IPI neurons and anxiety during nicotine withdrawal. ( a ) Representative photomicrographs from coronal sections containing the VTA (top). C57Bl/6J mouse brains were infected with control shRNA (ctrlRNA, left columns) or CRF shRNA (right columns) and were analysed for viral infection (green). Bottom, qRT-PCR comparing CRF (left) or TH (right) gene expression in ctrlRNA- and shRNA-infected VTA ( n =6 mice/group). Gene expression was normalized to GAPDH. *** P <0.001, two-tailed student’s t -test. ( b ) Top, photomicrographs depicting the IPI c-Fos pattern (green) induced by mecamylamine-precipitated withdrawal in chronic nicotine-treated mice expressing ctrlRNA (left) or CRF shRNA (right) in the VTA. Bottom, quantitative analysis of the number of IPI c-Fos immunopositive neurons during chronic nicotine before withdrawal and after mecamylamine-precipitated nicotine withdrawal from mice infected with ctrlRNA ( n =3 and 4 mice/group, 14 slices/mouse) or CRF shRNAs ( n =3 mice/group, 14 slices/mouse). ( c ) Top, photomicrographs depicting the IPR c-Fos pattern (green) induced by mecamylamine-precipitated withdrawal in chronic nicotine-treated mice expressing ctrlRNA (left) or CRF shRNA (right) in the VTA. Bottom, quantitative analysis of the number of IPR c-Fos immunopositive neurons during chronic nicotine before withdrawal and after mecamylamine-precipitated nicotine withdrawal from mice infected with ctrlRNA ( n =3 and 4 mice/group) or CRF shRNAs ( n =3). ( d ) Number of marbles buried in mice expressing ctrlRNA or CRF shRNA in the VTA during chronic nicotine exposure prior to withdrawal ( n =15 and 18, respectively) and during spontaneous nicotine withdrawal ( n =11 mice/group). ( e ) Time spent on the open arms of the EPM for mice expressing ctrlRNA or CRF shRNA in the VTA during chronic nicotine exposure prior to withdrawal ( n =15 and 20, respectively) and during spontaneous nicotine withdrawal ( n =11 mice/group). ( f ) Total arm entries in the EPM for each group in panel e . Data are expressed as mean±s.e.m. Scale Bar: 100 μm. Two-way ANOVA, Bonferroni post hoc test. ** P <0.01, ** P <0.001. ^ P <0.05, ^^ P <0.01 for between group comparisons. Full size image We compared anxiety-like behaviour in mice expressing shRNA and ctrlRNA in the VTA during chronic nicotine treatment and during spontaneous nicotine withdrawal. In the MBT, two-way ANOVA revealed a significant main effect of shRNA (F 1,51 =4.15, P =0.047), withdrawal state (F 1,51 =10.67, P =0.0019) and a significant interaction (F 1,51 =9.68, P =0.003). Mice expressing ctrlRNA buried significantly more marbles during withdrawal compared with mice receiving chronic nicotine ( Fig. 7d ). Conversely, shRNA-expressing mice did not increase their marble burying during spontaneous withdrawal compared with chronic nicotine-treated shRNA-expressing mice. In addition, shRNA-expressing withdrawn mice buried significantly less marbles than ctrlRNA withdrawn mice. Similarly, two-way ANOVA indicated a significant main effect of shRNA (F 1,53 =8.23, P =0.0059), withdrawal state (F 1,53 =8.91, P =0.0043) and a significant interaction (F 1,53 =5.66, P =0.021) in the EPM assay. CtrlRNA-expressing mice spent significantly less time in the open arms of the EPM during withdrawal compared with ctrlRNA mice receiving chronic nicotine ( Fig. 7e ). shRNA-expressing animals, on the other hand, spent similar times in the open arms regardless of withdrawal state. Withdrawn mice expressing shRNA spent significantly more time in the open arms of the EPM compared with ctrlRNA undergoing nicotine withdrawal. Neither shRNA nor withdrawal state significantly affected EPM total arm entries ( Fig. 7f ). These data indicate CRF synthesis in the VTA is critical for activation of the IPI during nicotine withdrawal, as well as withdrawal-induced anxiety. Here we show that the IPN is a brain region critical for the anxiogenic effects of nicotine withdrawal. Previous studies suggested a potential role of the Hb efferent pathways in modulating anxiety-like behaviour: lesioning the fasciculus retroflexus reduces anxiety-like behaviour on the EPM in rats, for example ref. 43 . In addition, a recent study ablated presumably glutamatergic neurons in the triangular septum, which innervate the MHb resulting in reduced anxiety-like behaviour in mice [44] . However, to our knowledge this is the first study implicating the IPN in the anxiogenic effects of nicotine withdrawal. Anxiety was induced during chronic nicotine exposure by an IPN infusion of mecamylamine, a non-specific nAChR antagonist used to precipitate nicotine withdrawal, in nicotine-dependent animals [11] , [45] . Previously, mecamylamine infusion into the IPN was shown to elicit physical withdrawal symptoms in nicotine-dependent animals through activation of GABAergic neurons in the IPR [22] . Thus, our data further implicate the IPN in affective nicotine withdrawal symptoms, but through a distinct subregion, the IPI. Interestingly, mecamylamine infusion into the IPN of nicotine-naive animals had little effect, indicating that chronic nicotine induces neuroadaptations in IPN efferents, or within the IPN itself, that increase sensitivity to nAChR blockade or nicotine cessation. Thus, when nAChR signalling is blocked or nicotine is removed after chronic exposure, there is a decrease in tonic activity of nAChRs, which triggers withdrawal. Confirming this idea, increased anxiety observed in mice undergoing spontaneous nicotine withdrawal was alleviated by an IPN infusion of nicotine. Future studies should focus on the nAChR subtypes involved in activation of the IPI during nicotine withdrawal. Previous studies implicated the extrahypothalamic stress system within the amygdala in negative emotional states, and anxiety during nicotine withdrawal [46] . Our data implicate the IPN as an additional component of the extrahypothalamic stress circuitry that is critical for nicotine withdrawal-induced anxiety. During nicotine withdrawal, neurons within a subregion of the IPN, the IPI, were activated. The IPI neurons activated during withdrawal express CRF1 receptors. Blockade of CRF1 receptors with a CRF1 receptor antagonist reduced activation of IPI neurons during nicotine withdrawal and also alleviated anxiety. In addition, infusion of CRF into the IPN was anxiogenic and reproduced the same selective pattern of IPI activation as that of nicotine withdrawal, suggesting CRF is released upon nicotine cessation thereby triggering anxiety. Activation of neurons through CRF1 receptor signalling is consistent with the ability of CRF1 receptors to potentiate the response of glutamate at AMPA/NMDA receptors [36] , [38] . Application of CRF to IPN slices elicited an increase in sEPSC amplitude and frequency consistent with both pre- and post-synaptic modulation of glutamatergic signalling through CRF receptors [47] . Importantly, we found that CRF potentiated evoked NMDA currents in IPI neurons and that reduction of glutamatergic signalling via an NMDA receptor antagonist reduced activation of IPI neurons during withdrawal while also alleviating anxiety. Interestingly, the IPN receives robust innervation from MHb cholinergic neurons, which also synthesize and release glutamate [48] . Optogenetic silencing of neurotransmission from cholinergic neurons of the MHb reduced activation of the IPI and anxiety during nicotine withdrawal, highlighting the critical role of glutamatergic input originating from dual cholinergic/glutamatergic MHb neurons. Recently, Grieder et al . [41] identified CRF synthesis in a unique population of VTA DAergic neurons as necessary for aversion and anxiety during nicotine withdrawal. In addition, CRF peptide density was reduced in the IPN of nicotine-withdrawn mice, consistent with CRF release in the IPN. Supporting this observation, our data indicate that a mesointerpeduncular circuit consisting of a population of VTA DAergic neurons projecting to the ventral IPN exists thereby providing a link between reward and aversion circuits. Knockdown of VTA CRF reduced activation of IPI neurons during nicotine withdrawal and prevented increased anxiety. Thus, the ventral IPN receives CRF input, at least partly, from VTA neurons. Our data identify a novel circuit and a mechanistic model for increased anxiety during nicotine withdrawal: chronic nicotine induces CRF synthesis in a population of VTA DAergic neurons that innervate the ventral IPN including the IPI. Chronic nicotine increases expression of the CRF1 receptor in Type II neurons of the IPI ( Fig. 8a ). During nicotine withdrawal, CRF from the VTA (and possibly other sources) is released thereby activating the upregulated CRF1 receptors on Type II IPI neurons and increasing pre- and/or post-synaptic glutamatergic signalling ( Fig. 8b ), which is dependent on MHb input. Ultimately, this increased glutamatergic input activates IPI neurons to trigger anxiety-like behaviours. Thus, the MHb and VTA converge onto the IPN to modulate anxiety. 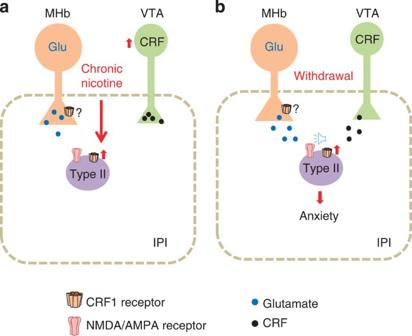Figure 8: Mechanistic model of increased anxiety during nicotine withdrawal. (a) The IPN receives glutamatergic input (Glu) from the MHb. Chronic nicotine induces CRF synthesis in a population of VTA DAergic neurons41that innervate the ventral IPN including the IPI. In addition, chronic nicotine increases expression of the CRF1 receptor in type II neurons of the IPI. (b) During nicotine withdrawal, CRF from the VTA is released and activates the upregulated CRF1 receptors on Type II IPI neurons, increasing signalling (speaker icon) and amplitude of sEPSCs (presumably through NMDA/AMPA receptors). CRF also increases sEPSC frequency indicating increased glutamate release, which stems from MHb inputs. We speculate that MHb terminals may also express the CRF1 receptor, which would underlie increased glutamate release during withdrawal. Figure 8: Mechanistic model of increased anxiety during nicotine withdrawal. ( a ) The IPN receives glutamatergic input (Glu) from the MHb. Chronic nicotine induces CRF synthesis in a population of VTA DAergic neurons [41] that innervate the ventral IPN including the IPI. In addition, chronic nicotine increases expression of the CRF1 receptor in type II neurons of the IPI. ( b ) During nicotine withdrawal, CRF from the VTA is released and activates the upregulated CRF1 receptors on Type II IPI neurons, increasing signalling (speaker icon) and amplitude of sEPSCs (presumably through NMDA/AMPA receptors). CRF also increases sEPSC frequency indicating increased glutamate release, which stems from MHb inputs. We speculate that MHb terminals may also express the CRF1 receptor, which would underlie increased glutamate release during withdrawal. Full size image Taken together, our data identify a novel circuit in addiction and implicate CRF1 receptors as therapeutic targets to facilitate smoking cessation by alleviating anxiety during nicotine withdrawal. Animals Male C57BL/6J, tyrosine hydroxylase (TH)-cre (Stock No. 00861) and choline acetyltransferase (ChAT)-cre (Stock No. 006410) mice were purchased from Jackson Labs, bred in the UMMS animal facility and used in behavioural, optogenetic and biophysical experiments as indicated. Animals (mice) were housed four/cage up until the start of each experiment. Animals were kept on a standard 12-h light/dark cycle with lights on at 0700 hours and off at 1900 hours. Mice were weaned at 21 days and were 6 weeks old at the start of chronic nicotine treatments. All experiments were conducted in accordance with the guidelines for care and use of laboratory animals provided by the National Research Council [49] , as well as with an approved animal protocol from the Institutional Animal Care and Use Committee of the University of Massachusetts Medical School. Drugs and drinking solution Nicotine and control drinking solutions were prepared from nicotine hydrogen tartrate or L -tartaric acid (Sigma-Aldrich), which were dissolved in tap water with the concentrations of 200 and 300 μg ml −1 , respectively. Saccharin sodium (Fisher Scientific) was added at a concentration of 3 mg ml −1 to each solution to sweeten the taste. Nicotine doses are reported as nicotine free base. For brain infusion, nicotine (50 ng μl −1 ), mecamylamine hydrochloride (2 μg μl −1 ), AP5 (0.2 μg μl −1 ), CRF (0.1 μg μl −1 , Sigma-Aldrich) and antisauvagine-30 (1 μg μl −1 , Tocris Bioscience) were dissolved in sterile saline. Antalarmin hydrochloride (Tocris Bioscience) was dissolved in 5% DMSO and 95% sterile saline (1 μg μl −1 ). Infusion concentrations and amounts for nicotine [50] , mecamylamine [11] , AP5 (refs 51 , 52 ), CRF [53] , antalarmin [54] and antisauvagine-30 (ref. 55 ) were chosen based on previously published studies. On the test day, the CRF1 antagonist antalarmin or the CRF2 antagonist antisauvagine-30 was administered 40 min before behavioural testing, while mecamylamine was administered 25 min before behavioural testing. CRF and nicotine were administered 10 min before behavioural testing. Lipophilic Tracer DiI (D282, Molecular Probe, Invitrogen, 5 mg ml −1 in ethanol) was used to locate the site of brain infusion. Cannula implantation For unilateral cannula implants, holes were drilled in the skull at the anteroposterior (AP, in reference to bregma) coordinates that correspond to IPN (−3.64 ∼ −3.80 mm AP), VTA (−3.28 ∼ −3.64 mm AP) or MnR (−4.04 ∼ −4.6 mm AP) based on the work of Paxinos and Franklin [56] . Stainless steel guide cannulas (26 gauge with 4 mm pedestals, Plastics One), with dummy cannulas in place, were inserted into the brain (−4.5 mm dorsal ventral for IPN or MnR and −4.25 mm for VTA) and secured to the skull with Cerebond (Plastics One). Mice were allowed to recover in individual cages for at least 3 days before behavioural testing. Intracerebral infusions Mice were anesthetized with 2% isoflurane via a nose cone adaptor at a flow rate of 800 ml l −1 . Once anesthetized, an infusion internal cannula (33 gauge) designed to reach 4.75 mm (for IPN and MnR) or 4.5 mm (VTA) below the skull was inserted into the guide cannula and vehicle, mecamylamine, CRF, AP5, antalarmin, antisauvagine-30 or nicotine was infused at a rate of 1 μl min −1 . After infusion, the cannula remained in position for 2 min before removal. Mice were placed back into their home cages and monitored until awake. After completion of behavioural experiments, mice were anesthetized, 1,1′-Dioctadecyl-3,3,3′,3′-Tetramethylindocarbocyanine Perchlorate (DiI) was infused, mice were culled and brains were removed and frozen on dry ice. Coronal sections (25 μm) were cut with a cryostat (Leica Microsystems, Inc.). Sections were mounted and stained with neutral red (Sigma) to visualize cannula placement and DiI infusion. From a total of 681 mice, 74 mice were excluded from analysis due to incorrect cannula placement. Exclusions were verified by an observer blinded to experimental groups. Immunohistochemistry For i.p. delivery of drugs, mice were given i.p. injections of saline daily for 3 days to habituate them to handling and to minimize neuron activation due to stress. During experiments, mice received a saline injection followed by another saline injection or received either a saline injection followed by a 3.0 mg kg −1 mecamylamine injection, or an injection of 10 mg kg −1 antalarmin followed by a 3.0 mg kg −1 mecamylamine injection as indicated. The time between the first and second injection was 15 min. Ninety minutes after the second injection, brains were removed and processed for immunolabeling. Mice were deeply anesthetized with sodium pentobarbital (200 mg kg −1 , i.p. ), perfused transcardially with 10 ml of ice-cold 0.1 M phosphate-buffered saline (PBS) followed by 10 ml ice-cold 4% (W/V) paraformaldehyde (PFA) dissolved in 0.1 M PBS (pH 7.4). Brains were removed and processed for immunolabeling as described previously [57] . Serial slices (25 μm) containing the IPN were collected between −3.28 and −3.88 mm from bregma. Rabbit anti-c-Fos (Santa Cruz, SC-52, 1:800) and rabbit anti-GAD1/2 (Sigma, G5163, 1:2,000) were used as primary antibodies to react with c-Fos and GAD1/2, respectively, while donkey anti-rabbit Alexa Fluor 488 (Life Technologies, A21207, 1:800) and donkey anti-rabbit Alexa Fluor 594 (Life Technologies, A11008, 1:800 ) were used as secondary antibodies. The number of c-Fos-immunopositive neurons was counted under a fluorescence microscope (Zeiss, Carl Zeiss MicroImmagine, Inc., NY, USA) at a magnification of 400 × . The intensity of fluorescence was quantified using a computer-associated image analyzer (Axiovision Rel., 4.6.1). Neurons were only counted as signal positive if intensities were at least two times higher than that of the average value of background. c-Fos-positive neurons were counted from all of the IPN serial slices, and the total numbers were compared between treatment and control. Combined CRF1 fluorescent in situ hybridization (FISH) and c-Fos immunohistochemistry Ninety minutes after CRF–IPN infusion, mice were anesthetized and transcardially perfused with 4% PFA as described previously. PFA was made with PBS DEPC-treated water. A digoxigenin (DIG) 5′- and 3′-labelled CRF1 LNA—enhanced oligonucleotide probe was synthesized by EXIQON (Exiqon, Inc.). An LNA mRNA detection control probe (ScrambleISH) was purchased from EXIQON as a negative control. Labelling was done using 30-μm thick free-floating brain sections. Following a PBS wash, sections were pretreated two times with saline sodium citrate buffer (SSC) for 25 min. Following DEPC water washes, sections were acetylated in 0.1 M triethanolamine (pH 8.0) for 1 min, then 0.25% (v/v) acetic anhydride for 10 min. Following washes in SSC, sections were dehydrated in a graded ethanol series (50, 70, 95 and 99%), each for 3 min. Hybridization was performed overnight at 54 °C in ISH buffer (Sigma-Aldrich) containing the probe (200 pmol). Post-hybridization washes included rinsing in SSC (4 × ), SSC (2 × ), SSC (0.5 × ) and SSC (0.1 × ), each for 30 min at 58 °C. Sections were then incubated in 3% H 2 O 2 for 15 min and PBS containing 0.1% Tween 20 for 3 min. Sections were then blocked for 1 h with PBS/0.3% Triton X-100/5% normal goat serum/1% BSA and incubated with anti-c-Fos primary antibody (1:800) overnight at 4 °C in blocking buffer. Following washes with 1 × PBS, sections were incubated with anti-DIG-FAB peroxidase (POD) antibody (Roche, 11207733910, 1:250) and goat anti-rabbit secondary antibody conjugated to Alexa Fluor 488 (1:800) to reveal the c-Fos signal for 2 h in a blocking solution containing 0.5% blocking reagent (Roche), 10% heat-inactivated goat serum and 0.1% Tween 20. Sections were then washed twice in PBS containing 0.1% Tween 20 followed by application of TSA Plus Cy3 (Perkin Elmer) for visualization of FISH. Slides were then washed three times in PBS, mounted onto Superfrost Plus slides and coverslipped with Vectashield mounting medium (Vector Laboratories). Images were taken using a fluorescence microscope at a magnification of 200 × or 630 × . IPN tissue collection and quantitative RT–PCR For collection of whole IPN tissue, brains were collected and placed on a glass slide and frozen on dry ice. Coronal sections ( ∼ 1 mm) were cut and the IPN was punched out using a Harris UNI-CORE (1.0 mm, Electron Microscopy Sciences). The cored IPN sample was transferred to a 1.5-ml collection tube containing lysis buffer. Laser Capture Microdissection (LCM) was performed to collect ventral IPN. The IPN serial sections were prepared as described previously [22] . Sections were fixed in ice-cold acetone followed by dehydration in a graded ethanol series. The Veritas Microdissection System Model 704 (Arcturus Bioscience, Inc.) was used for LCM. All ventral IPN areas were cut from each animal (from 50 slices per brain). Four mice were used per treatment. Neurons were captured on CapSure Macro LCM caps (Arcturus Bioscience, Inc.) and stored in 100 μl of lysis solution (Ambion). Total RNA was extracted from individual samples using a Micro Scale RNA Isolation Kit (Ambion). RNA samples extracted from the IPN were reverse-transcribed into cDNA using RT enzyme mix (20 × ) and RT buffer (2 × ; Ambion). PCRs were set up in 10-μl reaction volumes using TaqMan Gene Expression Assays (Applied Biosystems). Glyceraldehyde 3-phosphated dehydrogenase (GAPDH) was used as an internal control gene to normalize gene expression levels. PCR was performed using an ABI PRISM 7500 Sequence Detection System (Applied Biosystems). Negative controls with no reverse transcriptase were performed for all Taqman Assays. All reactions were performed in triplicate. Relative amplicon quantification was calculated as the difference between C t values of GAPDH and that of the gene of interest. Relative gene expression differences in IPN between nicotine-dependent mice and nicotine non-dependent mice were calculated using the 2 −ΔΔ C t method. Electrophysiology Brains were quickly removed and placed in oxygenated ice-cold high sucrose artificial cerebrospinal fluid containing kynurenic acid (1 mM, Sigma, St. Louis, MO, USA). Sucrose artificial cerebrospinal fluid solution contained (in mM): 250 sucrose, 2.5 KCl, 1.2 NaH 2 PO 4 ·H 2 O, 1.2 MgCl 2 ·6H 2 O, 2.4 CaCl 2 ·2H 2 O, 26 NaHCO 3 , 11 D -Glucose. Coronal brain slices containing IPN brain regions ( ∼ 180 μm) were made using a Leica VT1200 vibratome. Spontaneous EPSCs were obtained in the whole-cell configuration and gap-free acquisition mode in Clampex (Axon Instruments) as previously described [22] . Neurons were held at a resting membrane potential of −70 mV. For optical recordings, eYFP-positive neurons were identified under fluorescence microscopy. Trains of 593 nm (halorhodopsin, NpHR) or 470 nm (channelrhodopsin, ChR2) light pulses were applied to neurons under current clamp or voltage clamp using LEDs of the appropriate wavelength (Thor Labs), as indicated. Whole-cell NMDA currents in IPI neurons were evoked (duration of 100–200 μs, amplitude of 20–30 mA) by positioning a concentric bipolar electrode (FHC; Bowdoin, ME, USA) in an IPN region close to the IPI. NMDA currents were recorded while the membrane potential was held at +40 mV. Patch pipette solution for NMDA current recording contained the following (in mM): CsCH 3 SO 3 117, EGTA 0.4, NaCl 2.8, TEA-Cl 5, HEPES 20, Spermine 0.1, ATP 4, GTP 0.2. Evoked currents were recorded in the presence of CNQX (10 μM), in addition to bicuculline (20 μM) and atropine (1 μM). ACSF was used for bath solution and contained (in mM): 125 NaCl, 2.5 KCl, 1.2 NaH 2 PO 4 ·H 2 O, 1.2 MgCl 2 ·6H 2 O, 2.4 CaCl 2 ·2H 2 O, 26 NaHCO 3 , 11 D -Glucose. All recordings were filtered at 1 kHz using the amplifier’s four-pole, low-pass Bessel filter, digitized at 10 kHz with an Axon Digidata 1440A interface and stored on a personal computer. Spontaneous EPSCs were detected using Mini Analysis (Synaptosoft). Briefly, root mean square noise levels were measured to set an area threshold for rejecting noise events. The program was set to detect baseline from an average of 2 ms, 25–30 ms before the event peak and detect decay time based on the default 0.37 fraction of peak within 8 ms of the event. Multiplex and nested scRT–PCR At the end of each recording, the cytoplasm of individual neurons was aspirated into the recording pipette containing electrode solution made with DEPC-treated deionized water. RNA isolation, reverse transcription and amplification of CRF1 receptor mRNA was done as previously described [8] . Virus preparation Packaging of AAV-Ef1A-DIO-ChR2-eYFP plasmid, AAV-Ef1A-DIO-eNpHR3.0-eYFP and AAV-Pl-CMV-cre-ZsGreen (control virus) into AAV2 viral particles was done by the University of Massachusetts Medical School Viral Vector Core. AAV2 was used as the serotype for all viral-mediated gene deliveries as it has limited spread and thus, is well suited for focal infection into discrete brain regions [58] . For CRF silencing, Block-iT RNAi Designer (Life Technologies, Carlsbad, CA, USA) was used to select an shRNA sequence (shCRF, sense strand 5′-GGATCTCACCTTCCACCTTCT-3′) predicted to have high silencing efficiency. As a control, a ‘universal scramble’ shRNA with no homology to any transcripts was used (shSCR, sense strand 5′-GCGCTTAGCTGTAGGATTC-3′). Invitrogen Gateway technology was used to generate an AAV2 shuttle plasmid that encodes shCRF or shSCR downstream of the mU6 promoter and enhanced green fluorescent protein under the control of the cytomegalovirus (CMV) promoter 3′-flanked by a β-globin intron. Helper-free AAV2 particles were produced by the triple transfection of AAV-293 cells (Agilent Technologies Inc., Santa Clara, CA, USA) with the AAV2 shuttle plasmid described above, a plasmid that contains AAV2 rep and cap genes and a plasmid that encodes the adenovirus helper functions. Cells were collected and lysed by three freeze-thaw cycles, treated with benzonase and clarified by centrifugation 2 days after transfection. Viral vectors were purified and genomic units (GU) were quantified by RT–PCR. The titres were 4.5–6.6 × 10 11 GU ml −1 for shRNA virus and 3.0–8.5 × 10 12 GU ml −1 for opsin virus. Virus injection into MHb or VTA, and fibre optic cannula implantation Surgery and injections were performed as above and as described previously [22] . Halorhodopsin was injected into the MHb of ChAT-cre mice (0.5 μl per side). Mice were allowed to recover for at least 3 weeks before the start of experiments. After recovery, ChAT-cre mice were anesthetized and implanted with a fibre optic cannula in the IPN, consisting of a stainless steel ferrule, 1.25 mm in diameter with a 200-μm thick, 5-mm long cleaved flat optic fibre (Doric Lenses). Instant adhesive was placed between the base of the cannula and the skull, the scalp incision was stitched and dental cement was used to stabilize the cannula to the skull. Mice were allowed to recover in their home cages for at least 3 days before optic stimulation. ChR2 was injected bilaterally or unilaterally into the VTA of TH-cre mice (1 μl per side) for electrophysiology recording and VTA–IPN fluorescence imaging, respectively. shRNA of CRF or SCR RNA was bilaterally injected into the VTA (1 μl per side) and mice were allowed to recover in their home cages for at least 4 weeks before behaviour experiments or measuring of CRF expression in the VTA. In vivo optical silencing Infected ChAT-cre mice with stainless steel ferrule implants were gently connected to a patch cable using a mating sleeve (Doric Lenses). The optic fibre was attached through an FC/patch cable adaptor to a fibre-coupled LED light source. Yellow light pulses (593 nm) were generated through an LED driver. The light stimulation paradigm was continuous light pulses at 5 Hz with 500 mA current and 25% duty cycle. Light-on epochs were 35 min for all animals. Anxiety symptoms were recorded immediately after the first light pulse and were measured over the course of 30 min in the MBT assay and 5 min in the EPM assay. After recording, the ferrule was disconnected from the LED patch cable. Mice were euthanized and the brains were collected for analysis of virus injections and fibre implantations. A separate group of mice received a mecamylamine (1 mg kg −1 , i.p) injection immediately before the first light pulse and were kept in their home cages for another 55 min. Mice were anesthetized, perfused and the brains were removed for immunohistochemistry. Marble-burying test (MBT) All behaviours were measured during the light cycle. The assay consisted of placing 15 sterilized 1.5-cm glass marbles evenly spaced in five rows of three, each 4 cm apart on a 5–6-cm layer of bedding in a standard mouse cage. A mouse was placed in its test cage and left for 30 min, then removed to its home cage, and the number of marbles buried with bedding (to 2/3 their depth) was counted. Mice were habituated in the test cage for 2 days (45 min per day) before the test. Elevated plus maze (EPM) The experimental apparatus consisted of a central axis (5 × 5 cm), four arms elevated 45 cm above the floor, with each arm positioned perpendicularly to the adjacent arms. Two closed arms were enclosed with high walls (30 × 5 × 15 cm) while the other arms were open (30 × 5 × 0.25 cm). One 60 W red fluorescent light located 100 cm above the maze was used as the source of illumination. The mice were individually placed in the center of the maze with their heads facing one of the open arms and allowed 5 min of free exploration. The number of entries into the open and closed arms and the total time spent in the open and closed arms were measured by MED-PC IV software (MED Associates, Inc.). The time spent in open and closed arms was calculated as standard anxiety indices. The total number of arm entries was considered as an index of locomotor activity. The apparatus was cleaned thoroughly between trials. Mice that remained in the arm in which they were initially placed were not included in the analysis. Cotinine measurements The Cotinine Direct ELISA Kit (CalBiotech, Inc.) was used to measure cotinine in mouse blood serum according to the manufacturer’s instructions. Mice were exposed to nicotine or control solution at least 4 weeks before cotinine measurements. Blood for analysis was collected in the morning, 1 h after lights-on. Data analysis Data were analysed using one-way or two-way ANOVA followed by Bonferroni post hoc tests or two-tailed t -tests as indicated. Two-way ANOVA was used for mecamylamine-precipitated withdrawal experiments using mecamylamine/saline injection and chronic nicotine/control treatment as main factors. Two-way ANOVA was also used to analyze effects of IPN infusions on withdrawal behaviours with infusions and chronic treatment as main factors. One-way ANOVA with repeated measures was used to analyse effects of CRF drugs on sEPSC data. Two-tailed t -tests were used for analysis of chronic treatment on gene expression. Each data set was tested for normal distribution before analysis. Animal numbers were determined based on previous studies with similar endpoints [11] , [22] . Behaviour and immunohistochemistry data were analysed using GraphPad software. How to cite this article: Zhao-Shea, R. et al . Increased CRF signalling in a ventral tegmental area-interpeduncular nucleus-medial habenula circuit induces anxiety during nicotine withdrawal. Nat. Commun . 6:6770 doi: 10.1038/ncomms7770 (2015).